Pure second harmonic current-phase relation in spin-filter Josephson junctions Higher harmonics in current-phase relations of Josephson Junctions are predicted to be observed when the first harmonic is suppressed. Conventional theoretical models predict higher harmonics to be extremely sensitive to changes in barrier thickness, temperature, and so on. Here we report experiments with Josephson junctions incorporating a spin-dependent tunnelling barrier, revealing a current-phase relation for highly spin polarized barriers that is purely second harmonic in nature and is insensitive to changes in barrier thickness. This observation implies that the standard theory of Cooper pair transport through tunnelling barriers is not applicable for spin-dependent tunnelling barriers. The supercurrent through a Josephson junction (JJ) is conventionally described by means of a current-phase relation (CPR) I = I c sin φ where I c is the critical current and φ is the junction phase-difference. More generally, the CPR can be expressed as [1] , [2] and under circumstances in which the first harmonic is suppressed (for example at a 0–π transition), the second harmonic may become detectable [3] , [4] . Recently it has been predicted that, in JJs with diffusive ferromagnetic barriers and asymmetric spin-active interfaces, the CPR should be inherently dominated by the second harmonic as a consequence of the coherent transport of two triplet pairs [5] , [6] , but no theoretical predictions of a similar nature exists for the tunnelling limit. A dominant second harmonic in the CPR can be manifested as half-integer Shapiro steps and magnetic interference patterns I c ( H ) with half the expected period [7] . While there have been experimental reports of half-integer Shapiro steps near to 0– π transitions in S/F/S JJs with both weak [3] and strong [4] diffusive F layers, evidence of a second harmonic in CPR has not been reported in I c ( H ) patterns, although the periodicity of I c ( H ) is the most unambiguous probe of CPR. Gadolinium nitride is one of the few known ferromagnetic insulators and has previously been shown by our group to yield high quality superconducting tunnel junctions when placed between NbN electrodes [8] ; normal-state measurements have demonstrated spin filter behaviour with high-spin polarization P (ref. 9 ) (For details of calculation of P please refer to Supplementary Fig. 1 and Supplementary Methods ). Here, we report measurements of tunnel junctions with ferromagnetic GdN barriers in which the period of the magnetic field modulation of I c ( H ) halves at the onset with thickness corresponding to a large spin polarization of the tunnelling. The devices reported here show a spin polarization exceeding 80%, which is higher than previously reported (for fabrication and measurement details see the Methods section). For the largest thicknesses, I c ( H ) tends to a perfect half-period Fraunhofer pattern corresponding to a pure second harmonic CPR [7] . Role of barrier magnetic flux Throughout the paper, we will be treating our devices as being in the short junction limit, as calculations of Josephson penetration depth λ J (for details of calculation of λ J , please refer to the Methods section) for all samples reported here reveal that the junction dimension is much shorter (for high barrier thickness (>2.1 nm) and low-current density samples) or at most, comparable (for lower thickness (1.5 nm), higher-current density non-magnetic GdN samples) to λ J . The I c ( H ) pattern of a short JJ with a magnetic barrier is distorted by the field-dependent flux arising from the barrier magnetism [10] and so analysis requires the magnetic state of the barrier to be understood. In Fig. 1 , we show typical I c ( H ) patterns of a GdN JJ with a high P (~89% at 4.2 K) where the sequence of applied fields is split into three stages for clarity. 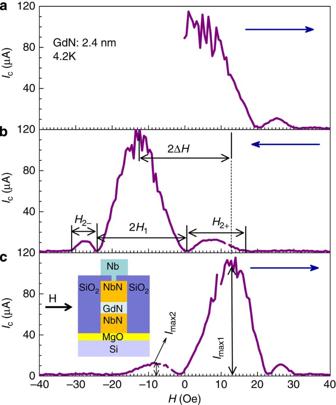Figure 1: DefiningIc(H) features of typical GdN junctions. Behaviour of critical current with externally applied in plane magnetic field broken into 3 parts showing the direction of field sweeps in each case. (a) Initial sequence of increasing external magnetic field analogous to virgin curve of correspondingMHloop. (b) Decreasing external magnetic field from positive to negative values. (c) Increasing external magnetic field from negative to positive values. ΔHis the hysteresis,H1is the magnitude of first lobe,H2+is the second lobe magnitude obtained after saturation of GdN,H2−is second lobe magnitude with the effect of micro-magnetics,Imax1andImax2are the maximum critical currents in the first lobe and second lobes respectively. Inset tocshows a schematic of cross section of a particular device with the direction of externally applied magnetic field. Figure 1a shows the initial field application sequence, which corresponds to the virgin curve of the corresponding GdN magnetization hysteresis loop M ( H ), in which the initially unmagnetized GdN layer is saturated by subjecting it to higher magnetic fields. Figure 1b shows the behaviour of the critical current when the field is reduced from positive to negative saturation fields and Fig. 1c shows the return branch to positive saturation. Several features are observed in Fig. 1 that are distinctly different from I c ( H ) patterns of conventional short JJs. First, the role of field history is evident as the maximum critical current of the central, or first, lobe is hysteretically shifted from zero field in Fig. 1b,c , indicating that the flux arising from the magnetic moment of the GdN barrier needs to be offset by an externally applied field in order to obtain the zero-flux maximum I c (ref. 10 ). Second, the ratio I max2 / I max1 is significantly lower than the value of 0.21 expected for a conventional Fraunhofer I = I c |sin x / x | dependence. This indicates the relative suppression of I c in the second lobe; a feature that was noted earlier [8] and was attributed to enhancement of the pair current in domain walls owing to large area devices. Finally, the field widths of the lobes of the I c ( H ) pattern are not constant so that H 2+ ≠ H 2− ≠ H 1 . These distortions from the behaviour expected for a perfect Fraunhofer pattern are due to the fact that thin film GdN has a low coercivity of 20–50 Oe (ref. 9 ) and because of their large area, our devices have multiple magnetic domains, and micromagnetic structure plays an important role in multidomain devices in distorting the I c ( H ) patterns [10] , especially in the switching regions. Because GdN has a high remnant moment, the second lobe in Fig. 1b marked as H 2+ , or its equivalent on the negative field side in Fig. 1c should be least distorted by the changes in flux arising from the barrier micromagnetics. Figure 1: Defining I c ( H ) features of typical GdN junctions. Behaviour of critical current with externally applied in plane magnetic field broken into 3 parts showing the direction of field sweeps in each case. ( a ) Initial sequence of increasing external magnetic field analogous to virgin curve of corresponding MH loop. ( b ) Decreasing external magnetic field from positive to negative values. ( c ) Increasing external magnetic field from negative to positive values. Δ H is the hysteresis, H 1 is the magnitude of first lobe, H 2+ is the second lobe magnitude obtained after saturation of GdN, H 2− is second lobe magnitude with the effect of micro-magnetics, I max1 and I max2 are the maximum critical currents in the first lobe and second lobes respectively. Inset to c shows a schematic of cross section of a particular device with the direction of externally applied magnetic field. Full size image In order to assess the extent of any such distortion, we model the field dependence of the magnetic moment of a hysteresis loop of GdN by a function where is the saturation moment of the GdN at a particular temperature and b , c , k are fitting parameters. A fit to a measured MH loop using this function is provided in Supplementary Fig. 2 . For magnetic barriers, since the barrier magnetic moment couples with the externally applied magnetic field, the relation for critical current variation with magnetic field can be expressed as: Where the flux quantum Φ 0 =2.06783461 × 10 −7 Gcm 2 , Φ B is the flux due to barrier moment, Φ is flux due to externally applied magnetic field, H is the externally applied magnetic field in Gauss, F is the magnitude of magnetic field corresponding to one flux quantum for a particular device geometry, d is the thickness of GdN layer and L is the length of device edge perpendicular to magnetic field. All calculations are done in CGS units. 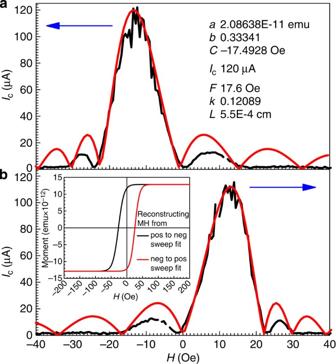Figure 2: Role of barrier flux in distortion ofIc(H). Fit to data ofFig. 1b,cusing the expressions derived in the text that takes into account the role of barrier magnetism inIc(H) patterns. (a) Fit for positive–to–negative field sweep. (b) Fit for negative-to-positive field sweep. The matching fits in the horizontal axes agrees with our assumption that barrier magnetism distorts the patterns from their conventional Fraunhofer-type shapes and thatH2+is least distorted due to magnetic effects. Inset shows the reconstruction of M-H loops of the device area of GdN, the parameters for which are obtained from the values used for fitting theIC(H) patterns. Figure 2 shows the fitting performed on data presented in Fig. 1b,c by using the above-mentioned equations. It is evident that the second lobe on the positive axes during the positive–to-negative field sweep (or second lobe on negative field axes during negative-to-positive field sweep) is least distorted. From the fits shown above, we find that when compared with the expected lobe size ( F ), H 2+ shows a distortion of only about 5%, whereas H 1 and particularly H 2− are distorted considerably more. Thus, we use the experimentally obtained values of H 2+ as the most reliable measure of period of I c ( H ). Figure 2: Role of barrier flux in distortion of I c ( H ). Fit to data of Fig. 1b,c using the expressions derived in the text that takes into account the role of barrier magnetism in I c ( H ) patterns. ( a ) Fit for positive–to–negative field sweep. ( b ) Fit for negative-to-positive field sweep. The matching fits in the horizontal axes agrees with our assumption that barrier magnetism distorts the patterns from their conventional Fraunhofer-type shapes and that H 2+ is least distorted due to magnetic effects. Inset shows the reconstruction of M-H loops of the device area of GdN, the parameters for which are obtained from the values used for fitting the I C ( H ) patterns. Full size image Comparison with non-magnetic junctions In Fig. 3 , we compare I c ( H ) patterns of magnetic and non-magnetic junctions. NbN/MgO/NbN junctions and NbN/GdN/NbN junctions with a non-magnetic GdN (low thickness of GdN barrier, equivalent to dead layer thickness) have almost identical characteristics expected of a dependence, where Φ 0 is the flux quantum, Φ is the flux arising due to externally applied magnetic field. It is evident that the various parameters defined in Fig. 1 in order to characterize the I c ( H ) patterns are strongly affected by increasing the GdN barrier thickness, which in turn increases the barrier magnetism and P . Representative IV characteristics of magnetic and non-magnetic GdN junctions are shown in Supplementary Fig. 4 . I c ( H ) patterns of a series of MgO junctions are shown in Supplementary Fig. 5 to demonstrate that the data used in Fig. 3a are representative of general characteristic of NbN/MgO/NbN JJs. 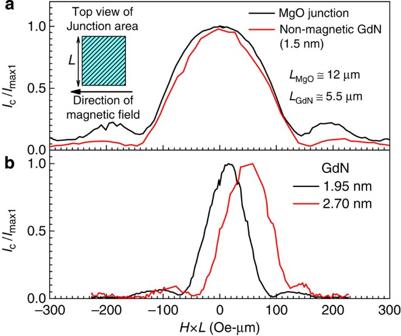Figure 3: Comparison ofIc(H) patterns with non-magnetic junctions. Comparison of non-magnetic GdN JJs with MgO JJs and demonstrating the evolution of magnetic GdN barrier JJs with thickness (a) NbN/MgO/NbN junction of different geometry compared with a non-magnetic GdN junction, to establish that the low thickness non-magnetic GdN and a non-magnetic insulator are similar. (b) Magnetic interference patterns of JJs with two different thickness of GdN layer, which demonstrate how parameters described inFig. 1evolve with increasing GdN thickness. The observed differences in characteristics ofIc(H) patterns can thus be attributed to magnetism of GdN barrier. Figure 3: Comparison of I c ( H ) patterns with non-magnetic junctions. Comparison of non-magnetic GdN JJs with MgO JJs and demonstrating the evolution of magnetic GdN barrier JJs with thickness ( a ) NbN/MgO/NbN junction of different geometry compared with a non-magnetic GdN junction, to establish that the low thickness non-magnetic GdN and a non-magnetic insulator are similar. ( b ) Magnetic interference patterns of JJs with two different thickness of GdN layer, which demonstrate how parameters described in Fig. 1 evolve with increasing GdN thickness. The observed differences in characteristics of I c ( H ) patterns can thus be attributed to magnetism of GdN barrier. Full size image Thickness dependence of junction parameters In Fig. 4 , we plot various junction parameters as a function of GdN thickness. Most data points are averages of at least four junctions of the same barrier thickness and the error bars indicate the spread of values. The critical current is measurable up to a thickness of 2.9 nm but the second lobe in the I c ( H ) patterns is undetectable above 2.7 nm. 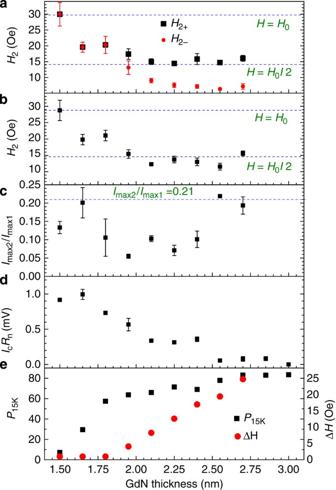Figure 4: Thickness dependence of junction parameters. (a) Magnitude of second lobesH2on either side; (b) magnitude of first lobeH1; (c) ratio ofImax2/Imax1(d)IcRnproduct; (e) hysteresis inIc(H) and spin polarization at 15 K. Figure 4: Thickness dependence of junction parameters. ( a ) Magnitude of second lobes H 2 on either side; ( b ) magnitude of first lobe H 1 ; ( c ) ratio of I max2 / I max1 ( d ) I c R n product; ( e ) hysteresis in I c ( H ) and spin polarization at 15 K. Full size image The primary results of this paper are reported in Fig. 4a,b , which shows the changes in the I c ( H ) lobe width with GdN thickness. The lines labelled H 0 in Fig. 4a,b are derived from all the non-magnetic junctions in our study. Since the thickness of our superconducting NbN layers are less than the London penetration depth ( λ ) of NbN (200–250 nm at 4.2 K), the expression for external field required for first minimum in I c ( H ) is [11] , [12] , [13] : From λ values reported in the literature (200–250 nm), and L (5.5–7 μm) obtained by measuring junction dimensions after fabrication, and NbN film thickness d F =100±10 nm, we therefore estimate H 0 =33.4±4 Oe. The experimental data from the non-magnetic junctions (left most point in Fig. 4a,b ), matches very closely with this estimate. The NbN electrodes are of identical thickness for all samples, the device dimensions are constant in all devices and hence, H 1 and H 2+ should be equal to H 0 regardless of the GdN thickness. However, it is evident that for the junctions in which the magnetism and spin polarization are well developed, H 1 and H 2+ converge rapidly to a value of H 0 /2 once magnetism is established. Because the other junction parameters are fixed, this observed decrease in H 1 and H 2+ therefore has a more fundamental origin. Earlier it was argued that H 2+ gives the most accurate estimate of the undistorted magnitude of the I c ( H ) lobes, and it is clear from the data that the deviation from H 0 /2 is less than 10%; that is, for fully magnetic barriers the I c ( H ) patterns evolve to have exactly half the period expected from a conventional I = I c |sin x / x | relation; a behaviour expected of junctions that have CPR dominated by second harmonic [7] , [14] . An identical trend is found for behaviour of H 1 albeit with a somewhat larger scatter arising from the distorting effects arising from the reversal of GdN magnetism. Once established, this halving of the period is independent of GdN thickness; in contrast, H 2− lies in the field region in which the barrier moment is switching and so, with increasing barrier thickness, H 2− is progressively reduced as shown in Fig. 4a . This interpretation of second harmonic-dominated CPR for the most magnetic barriers is supported by the data in Fig. 4c , where the ratio of I max2 / I max1 initially decreases from the value of 0.21 expected for the standard Fraunhofer pattern as the magnetism turns on and recovers again ~0.21 for the most magnetic barriers implying that, provided the hysteretic effect of the barrier flux is accounted for, these junctions show ideal half-period I c ( H ) patterns as predicted elsewhere [7] . We have attempted to measure Shapiro steps in these devices, but have been unable to resolve them with sufficient detail to provide any additional information. The hysteresis (Δ H ) in I c ( H ) shown in Fig. 4e increases linearly with thickness as expected if the barrier moment couples directly with the externally applied magnetic field. The spin polarization at 15 K ( P 15 K ) shown in Fig. 4e shows a similar trend with thickness as observed previously [9] . Our results provide direct evidence for a pure second harmonic in the current-phase relation of NbN/GdN/NbN devices for all barrier thicknesses greater than 2 nm. Since the second harmonic in our devices is independent of barrier thickness and in the sense originally introduced by Trifunovic [5] , the dominance of the second harmonic is ‘robust’; meaning its origin cannot be explained on the basis that the devices are at or near 0– π transitions, as such regions are limited to narrow and specific barrier thickness [15] . Therefore, the dominance of the second harmonic reported here must have a more fundamental origin. The most relevant theoretical studies [16] , [17] of spin-filter JJs consider first-order tunnelling processes and take into account barriers with high-spin polarization and asymmetry of exchange fields in the superconducting electrodes induced by the ferromagnetic barrier [18] . Under conditions of high-spin polarization and where the exchange field is of equal magnitude but different direction in the two electrodes, these studies predict a triplet component of the supercurrent. Although developed for very different systems (junctions with a sufficiently thick metallic ferromagnet barrier such that the singlet supercurrent is blocked), the existing theories that predict a robust dominant second harmonic depend on an asymmetry in the interfacial magnetic inhomogeneity, which generates the triplet pairs-specifically that a spin-active interface exists only at one side of the barrier such that the coherent transport of two spin triplet pairs are required to carry a supercurrent. By combining these two pictures, we can obtain a possible qualitative picture of the origin of the dominant second harmonic term in our devices. First, the quasiparticle conductance spectra [19] of our devices are strongly asymmetric in voltage, which implies [18] a difference in the exchange fields induced in the two electrodes (please refer to Supplementary Fig. 6 and Supplementary Note 1 ), and hence there potentially is only one spin-active interface that could give rise to higher-order tunnelling processes. Second, the data in Fig. 4e show that second harmonic appears at fairly high-spin polarization that favours triplet pair transmission over singlet. Nevertheless, it should be noted that the I c R n product decreases rapidly with increasing spin polarization ( Fig. 4d ), which is not expected for first-order triplet tunnelling [16] , but such decrease of amplitude of robust second harmonic component of CPR (consisting of opposite spin triplet pairs) is predicted for high-spin polarizations [6] . This observation leads to the suggestion that, in our devices, higher-order tunnelling processes, which generate two triplet pairs, are playing a dominant role in the generation of second harmonic CPR. In the absence of an adequate theory of higher order tunnelling in spin-filter Josephson junctions, it is not possible to provide greater certainty as to the origin of dominant second harmonic in our devices; however, our results demonstrate that for barriers with high-spin polarization, the period of Fraunhofer patterns is halved, and higher-order tunnelling processes might be at play in a spin-filter JJ, which can lead to higher harmonics in CPR. Film growth and junction fabrication The NbN/GdN/NbN films were grown on oxidized Si substrates precoated with a 10-nm-thick layer of MgO; the MgO layer protects the oxidized Si during fabrication by acting as an etch stop layer while etching NbN with CF 4 , and serves no other purpose in device function. The thicknesses of the top and bottom NbN layers were 90 and 100 nm respectively. NbN and GdN films were deposited by reactive d.c. sputtering in an Ar/N 2 atmosphere from pure Nb and Gd metal targets in an ultra-high vacuum chamber without breaking the vacuum. Multiple substrates were rotated at differing speeds below a stationary Gd target using a computer-controlled stepper-motor in order to obtain samples with different GdN barrier thicknesses in the same deposition run. The MgO barrier was deposited by radio frequency sputtering from an MgO target in pure argon, followed by a post-deposition r.f. plasma oxidation stage. Mesa tunnel junctions were then fabricated using a four-stage lithography process. Transport measurements Fabricated junctions were measured by a four-point current bias technique using a dip probe in a liquid helium dewar. A solenoid was used to apply in-plane magnetic fields. The sample space was shielded from external stray fields by means of a μ-metal shield. Magnetic measurements of thin film GdN Magnetic measurements of thin film GdN were done using films of AlN/GdN/AlN in order to eliminate diamagnetic signal that would have risen from superconducting NbN films. The top and bottom layers of AlN are deposited to ensure that GdN does not react with atmosphere and substrate, respectively. Josephson length λ J The Josephson length λ J is calculated using the expression , where for non-magnetic junctions (ref. 11 ) and for magnetic junctions (ref. 20 ), where μ r is the relative permeability of GdN. We estimate the permeability via μ r =1+ χ , where χ is the susceptibility obtained by fitting a straight line at the switching region of magnetic moment of M-H loop as shown in Supplementary Fig. 3 (we should note that this is likely to overestimate the small-signal μ r , which is relevant for the calculation of λ J ). Although χ will vary with applied magnetic field, the highest values of χ should be in the switching regions (in the switching regions χ =84 whereas by fitting a straight line to the low field M-H behaviour of the virgin curve, we obtain χ =61). Again, we use the highest possible value of χ to get the lowest estimate of λ J to compare with the junction dimension L. For the non-magnetic junctions of the same deposition run as the magnetic samples, with d=1.5 nm of GdN (average critical current density J c =6.73 × 10 6 Am −2 ), λ J =6.2±0.9 μm. This is approximately equal to L and is therefore the junction is more or less in the short junction limit. For non-magnetic junctions from other runs, whose data are included in the left-most point of Fig. 4a of the manuscript the current density is lower and therefore more firmly in short junction limit. As discussed above, our measured values of H 0 for these devices agree with the calculated values now provided and so the possibility of distortion by long-junction effects can be eliminated. From the magnetic junctions presented in Fig. 4 , the highest J c for junctions with H 2+ ≅ H 0 /2 is the sample with d =2.1 nm of GdN. For that sample (average J c =2.73 × 10 6 Am −2 ), λ J =8.9±1 μm is considerably more than the junction dimension L . For the sample with lowest current density with d =2.8 nm of GdN (average J c =5.37 × 10 5 Am −2 ), λ J =20±3 μm. Hence, all magnetic junctions are in the short junction limit. How to cite this article : Pal, A. et al. Pure second harmonic current-phase relation in spin-filter Josephson junctions. Nat. Commun. 5:3340 doi: 10.1038/ncomms4340 (2014).